Fast low-voltage electroactive actuators using nanostructured polymer electrolytes Electroactive actuators have received enormous interest for a variety of biomimetic technologies ranging from robotics and microsensors to artificial muscles. Major challenges towards practically viable actuators are the achievement of large electromechanical deformation, fast switching response, low operating voltage and durable operation. Here we report a new electroactive actuator composed of self-assembled sulphonated block copolymers and ionic liquids. The new actuator demonstrated improvements in actuation properties over other polymer actuators reported earlier, large generated strain (up to 4%) without any signs of back relaxation. In particular, the millimetre-scale displacements obtained for the actuators, with rapid response (<1 s) at sub-1-V conditions over 13,500 cycles in air, have not been previously reported in the literature. The key to success stems from the evolution of the unique hexagonal structure of the polymer layer with domain size gradients beneath the cathode during actuation, which promotes the bending motion of the actuators. Recently, electroactive actuators that show reversible mechanical deformation in response to an electric field have received enormous interest in the era of biomimetic technology, including robotics [1] , microsensors [2] and artificial muscles [3] , [4] . In particular, ionic polymer actuators, which are a category of electroactive actuators, comprising a layer of polymer electrolyte sandwiched in between electrodes have emerged as promising candidates in such applications, owing to their lightweight, flexibility, mechanical robustness and ease of fabrication at low cost [5] , [6] , [7] . As the electromechanical motion in ionic polymer actuators occurs through the migration of ions towards oppositely charged electrodes upon the application of an electric field [8] , [9] , ion transport properties and electrochemical stability of polymer electrolytes have important roles in determining the performance of the actuators [10] , [11] . Conventional polymers that appear to be leading candidates for the actuators include poly(vinylidene fluoride) (PVdF)-based polymers [12] , [13] , [14] , [15] , conjugated polymers [16] , [17] and perfluorinated ionomers with random inclusions of acidic moieties (that is, Nafion) [18] , [19] , [20] . To facilitate actuation response to a given voltage, additional solvents have typically been incorporated in these polymers [21] . The most important requisites for the ionic polymer actuators are large displacements in bending motion, fast switching response, low operating voltage, and durable operation in air [14] , [15] , [22] , [23] . Current ionic polymer actuators are yet short of the requirements, especially because of the slow actuation response and drastically reduced displacements under low-voltage operation [24] . A large number of actuators have also revealed the inherent drawback of a limited electrochemical stability window of the applied voltage, which is intimately linked to the physicochemical instability of additive molecules, leading to deterioration of performance with prolonged operation [25] . The above requirements and challenges have spurred researches to utilize ionic liquids in the actuators [13] , [22] , [25] , [26] because of their fascinating characteristics of negligible vapour pressure, high ionic conductivity and a large electrochemical stability window [27] , [28] . The use of ionic liquids resulted in improved actuation performance in a wide window of applied voltage [15] , [29] , which was attributed to effective swelling at the cathode and shrinkage at the anode as a result of the migration of cations and anions dissociated from the ionic liquids. The reliable response of the actuators in air is also achieved with the utilization of hydrophobic ionic liquids by reducing the tendency to absorb water [30] , [31] . To design ionic liquid-containing polymer electrolytes that suit the actuators, recent studies have concentrated on the application of a range of ionic liquids, taking into account the different van der Waals’ volumes of cations and anions, and the concentration polarization derived from dissimilar diffusivities of the cations and anions [25] , [29] , [32] . Although the introduction of ionic liquids has led to outstanding progress in the field of ionic polymer actuators, less attention has been paid to the exploitation of a new polymer [23] , [33] , [34] , [35] . In fact, research on actuators comprising ionic liquids has commonly used a few conventional polymers [25] , [26] , thus impeding major advances in ionic polymer actuators, which essentially require the optimization of ion transport characteristics and mechanical properties of the polymer layer. In this respect, the use of microphase-separated polymers in actuators has recently been proposed as a promising means to elevate the actuator performance [7] , [10] , [33] , [34] , [35] , [36] , [37] , [38] , [39] , [40] , [41] . For instance, Long et al. [34] , [35] , Spontak et al. [7] , [36] , [37] , Colby et al. [38] , [39] and Watanabe et al. [10] , [40] , have employed self-assembled block copolymers in actuators and improved electromechanical deformation has been reported, compared with that of several conventional polymers lacking organization. Although this is intriguing, it should be noted here that the actuators composed of nanostructured polymer electrolytes still have deficiencies in their properties when compared with the best results obtained with state-of-the-art polymers that possess ill-defined morphologies, namely PVdF [41] and PVdF derivatives [42] . In particular, there has been no substantial progress in lowering the operation voltage of the actuators. This implies that information on how the nanoscale ionic channels in the polymer layer influence the switching response and bending motion of the actuators is necessary to identify the role of self-assembled polymer electrolytes in determining actuator properties that should be targeted for further improvement. In the present study, we are motivated to develop a new ionic polymer actuator comprising nanostructured sulphonated block copolymers and ionic liquids with a tailored degree of ionic interaction. Our actuator exhibits much better actuator performance than previously reported ionic polymer actuators. These characteristics are intimately related to the fast and organized ion motion along the well-connected ionic channels within the self-assembled polymer layer. The main aim of this study is to propose a platform to advance the performance of ionic polymer actuators by clarifying the role of polymer electrolyte layers. We focus especially on the development of low-voltage-driven actuators with the goal to build biomimetic actuators with human affinity applications that are operable over a long period of time with a small battery. The new actuator developed is capable of millimetre-scale displacements with sub-1-V actuation, which is a new record in polymer actuators. We believe that our results can lead to the design of new polymers to offer unprecedented access to next-generation electromechanical devices. Morphology of block copolymers containing ionic liquids The molecular structure of poly(styrenesulphonate-b-methylbutylene) (PSS-b-PMB) block copolymers is shown in Fig. 1a . The covalently bonded non-ionic PMB chains are intended to retain the mechanical integrity with the incorporation of ionic liquids. The copolymer is referred to as P17(SL) by denoting the sulphonation level (SL) in parentheses, which was varied from 20 to 75 mol%. 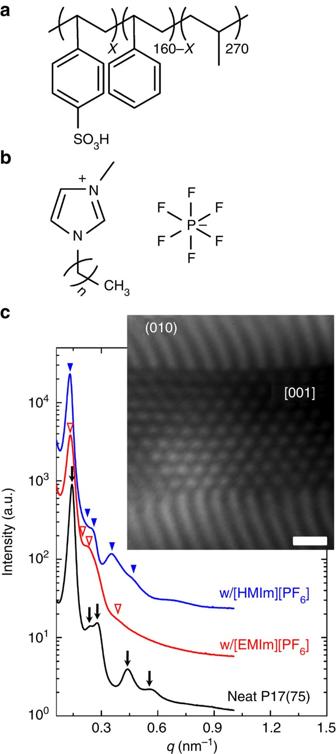Figure 1: Molecular structure and morphology. Molecular structures of (a) PSS-b-PMB block copolymer and (b) 1-alkyl-3-methyl imidazolium hexafluorophosphate. (c) SAXS profiles of P17(75) membranes with the addition of [HMIm][PF6] and [EMIm][PF6] at 25 °C. The arrows for neat P17(75), the inverted open triangles of P17(75) integrated with 60 wt% [EMIm][PF6] and the inverted filled triangles of P17(75) containing 60 wt% [HMIm][PF6] represent Bragg peaks at q*,q*,q*,q* andq* indicative of HEX morphology. The scattering profiles are vertically offset for clarity. A cross-sectional TEM image of neat P17(75) copolymer given in the inset figure ofcshows the (010) plane and the [001] view of the HEX structure. Scale bar, 100 nm; the PSS phases were darkened by RuO4staining. We found that the Young’s modulus of the PSS-b-PMB copolymer was affected by the SL value, as listed in Table 1 , and the P17(75) copolymer with the highest SL exhibited a modulus as high as 3.25 GPa. Note that the Young’s moduli of conventional sulphonated polymers are reported as 0.2–1 GPa (ref. 43 ). Figure 1: Molecular structure and morphology. Molecular structures of ( a ) PSS-b-PMB block copolymer and ( b ) 1-alkyl-3-methyl imidazolium hexafluorophosphate. ( c ) SAXS profiles of P17(75) membranes with the addition of [HMIm][PF 6 ] and [EMIm][PF 6 ] at 25 °C. The arrows for neat P17(75), the inverted open triangles of P17(75) integrated with 60 wt% [EMIm][PF 6 ] and the inverted filled triangles of P17(75) containing 60 wt% [HMIm][PF 6 ] represent Bragg peaks at q*, q*, q*, q* and q* indicative of HEX morphology. The scattering profiles are vertically offset for clarity. A cross-sectional TEM image of neat P17(75) copolymer given in the inset figure of c shows the (010) plane and the [001] view of the HEX structure. Scale bar, 100 nm; the PSS phases were darkened by RuO 4 staining. Full size image Table 1 Characteristics of sulphonated block copolymers and ionic liquids. Full size table Figure 1b shows the chemical structure of ionic liquids used in the present study. The hexafluorophosphate [PF 6 ] anion was chosen to offer reasonable air stability of the polymer electrolyte layers because of its hydrophobic characteristics. Two different alkyl imidazolium cations, that is, 1-ethyl-3-methylimidazolium ([EMIm], n =1) and 1-hexyl-3-methylimidazolium ([HMIm], n =5) were employed while maintaining the same [PF 6 ] anion, yielding dissimilar melting temperatures, van der Waals’ volumes and binding energies of ionic liquids, as summarized in Table 1 . The thermodynamic immiscibility between the ionic PSS and non-ionic PMB phases can create self-assembled morphology, which offers short ion diffusion pathways along the nanoscale ionic channels. The morphologies of the PSS-b-PMB copolymers in the presence and absence of ionic liquids were examined by combining small-angle X-ray scattering (SAXS) and transmission electron microscope (TEM) experiments. For brevity, we will only discuss representative data obtained from a subset of the samples listed in Table 1 . Figure 1c shows SAXS profiles measured at 25 °C obtained from P17(75) copolymers integrated with different ionic liquids, compared with that of neat P17(75) copolymer. We observed a series of Bragg peaks (↓) at 1q*, q*, q*, q* and q*, with q *=2π/ d 100 and d 100 =43.6 nm for the neat P17(75) copolymer, indicating the formation of a well-defined hexagonal-cylindrical (HEX) morphology. When 60 wt% of [EMIm][PF 6 ] and [HMIm][PF 6 ] were added to the HEX-forming P17(75) copolymer, qualitatively similar Bragg peaks were observed for both samples, indicating non-significant changes in the HEX morphology. With [HMIm][PF 6 ], however, a relatively larger domain size of 47.8 nm was seen, compared with a value of 45.9 nm obtained with the use of [EMIm][PF 6 ]. Such dissimilar domain spacings were attributed to different van der Waals’ volumes of cations in ionic liquids, yielding a more effective swelling of ionic PSS domains upon incorporating [HMIm][PF 6 ]. It should also be noted that the analogous HEX morphology was observed for all samples with SLs in the range of 20–75 mol% and ionic liquid concentrations of 0–60 wt%. The HEX morphology was confirmed by cross-sectional TEM experiments on the cryomicrotomed membrane. The representative TEM image of P17(75) is shown in the inset figure of Fig. 1c , which provides the (010) plane and the [001] view of the well-defined HEX structure possessing non-ionic PMB cylinders dispersed in an ionic PSS matrix (the PSS phases were darkened by RuO 4 staining). The TEM result implies that the ion migration should be less interrupted by grain boundaries because of the intrinsically well-connected PSS phases, which was achieved by combining solvent casting and pressure-field alignment (details are given in Method section). The domain sizes obtained from the TEM images were in good agreement with the SAXS data. Performance of ionic polymer actuators We fabricated actuators consisting of single-walled carbon nanotube (SWCNT) electrodes and HEX-forming PSS-b-PMB block copolymers integrated with ionic liquids (details are given in Method section). Supplementary Fig. S1 shows a cross-sectional scanning electron microscope (SEM) image of the actuator with a monolithic trilaminar structure. 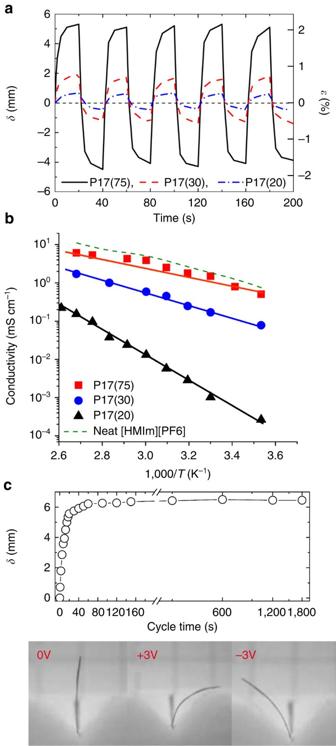Figure 2: Bending performance of actuators. (a) The displacement (strain) of the actuators comprising P17(20), P17(30) and P17(75) copolymers and 60 wt% [HMIm][PF6] at alternating square-wave voltages of±3 V and a frequency of 0.025 Hz. (b) Conductivities of P17(20), P17(30) and P17(75) membranes upon incorporating 60 wt% [HMIm][PF6]. The linear fits were obtained by Arrhenius plots. The conductivity of neat [HMIm][PF6] is shown by dotted line. (c) Time-dependent displacement of the actuator comprising P17(75) and 60 wt% [HMIm][PF6] at 3 V. Photographs taken at 120 s illustrate the equilibrium bending motion of the actuator at ±3 V. Figure 2a shows the time-dependent bending response of the actuators based on the P17(20), P17(30) and P17(75) copolymers, and [HMIm][PF 6 ] at alternating square-wave voltages of±3 V and a frequency of 0.025 Hz. The concentration of the ionic liquid was fixed at 60 wt% for all samples. The displacement ( δ ) was measured from the position of the actuator tip and a negative sign in the δ -value indicates that –3 V was applied to the actuator to yield the bending motion in the opposite direction. As can be seen from Fig. 2a , the largest average δ -value exceeding 5.2 mm (corresponding to ε =2%) was achieved with a cycle time of 20 s for the actuator composed of the ionic liquid-integrated P17(75) copolymer, whereas 1.7 mm and 0.6 mm were obtained with the use of P17(30) and P17(20) copolymers, respectively. Without doubt, we can conclude that the increased amount of –SO 3 H groups promoted the dissociation of ionic liquids, thereby offering the capability to improve the actuator performance by facilitating ion transport in the polymer layer [44] . The displacements obtained for different ionic liquid concentrations are presented in Supplementary Fig. S2 . When the concentration of ionic liquids is decreased from 60 to 45 wt%, we observed a twofold decrease in the generated strain at 3 V, as rationalized by the reduced amounts of active ions within the membranes. Figure 2: Bending performance of actuators. ( a ) The displacement (strain) of the actuators comprising P17(20), P17(30) and P17(75) copolymers and 60 wt% [HMIm][PF 6 ] at alternating square-wave voltages of±3 V and a frequency of 0.025 Hz. ( b ) Conductivities of P17(20), P17(30) and P17(75) membranes upon incorporating 60 wt% [HMIm][PF 6 ]. The linear fits were obtained by Arrhenius plots. The conductivity of neat [HMIm][PF 6 ] is shown by dotted line. ( c ) Time-dependent displacement of the actuator comprising P17(75) and 60 wt% [HMIm][PF 6 ] at 3 V. Photographs taken at 120 s illustrate the equilibrium bending motion of the actuator at ±3 V. Full size image The SL-dependent displacement was understood on the basis of dissimilar conductivities of P17(20), P17(30) and P17(75) copolymers upon incorporating the same amount of [HMIm] [PF 6 ] (60 wt%). As shown in Fig. 2b , the conductivity closest to that of neat ionic liquid was obtained for P17(75), which was responsible for the high electromechanical deformation. On the contrary, the conductivity was reduced by a few orders of magnitude for P17(20), where the value was significantly lower than that obtained for P17(30), implying that conductivity is not proportional to the SL value of the copolymers. We could infer that a threshold SL value existed for the formation of cocontinuous ionic channels within the PSS domains [45] , which could be located between 20 and 30 mol% for our samples. Below the threshold value, the efficiency of net ion transport appeared to be largely diminished, which eventually reduced actuation response. The total charge at the PSS-b-PMB copolymer integrated with [HMIm][PF 6 ] was the highest at 0.12 F g −1 for P17(75), followed by 0.025 F g −1 for P17(30) and 0.0078 F g −1 for P17(20), as determined from the capacitance measurements. Using the best performing actuator containing P17(75) and [HMIm][PF 6 ], we examined the time-dependent bending motion by applying a voltage of 3 V. This analysis assured durable response of the actuator by providing sufficient time for the ion migration. As shown in the plot in Fig. 2c , the initial time to respond to the actuation field was as short as 1 s where the movement was gradually suspended at around 20 s. Notably, no back relaxation was detected for an extended interval of up to 1,800 s, which is known as one of the common drawbacks of conventional actuators that limit the frequency range and accuracy of the actuator’s motion control [25] , [35] . This implies that the diffusion of [PF6] anions within nanoscale PSS domains is also fast as that of [HMIm] cations upon applying the actuation field and, thus, the back diffusion with extended actuation time is not taking place. Photographs taken at 120 s, as shown in Fig. 2c illustrate the equilibrium bending motion of the actuator at ±3 V. Factors affecting the actuation performance We now elucidate factors affecting the actuation performance beyond the SL of PSS-b-PMB copolymers. For most ionic polymer actuators, a large reduction in the generated strain is observed with the increase in frequency, the decrease in voltage of the activation field, or both, which hampers their use in practical applications [29] . This reduction primarily originates from the low ion mobility in the polymer layers. One noteworthy difference between our actuators and others’ reported in literatures is the markedly improved functionality of our actuators at high-frequency (>0.1 Hz) and low-voltage (1 V) conditions. 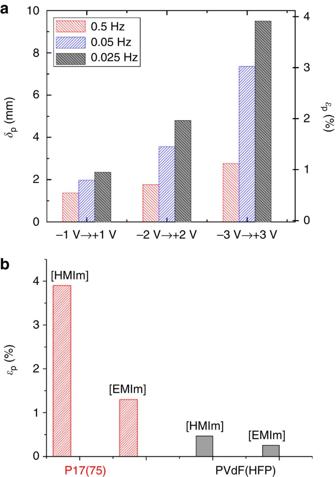Figure 3: Factors affecting the actuation performance. (a) Displacement (strain)-frequency-voltage dependency of the actuator comprising P17(75) and [HMIm][PF6] measured with alternating square-wave voltages. (b) Peak-to-peak strain values of the actuators comprising P17(75) and ionic liquids, compared with those of PVdF-HFP and ionic liquids, by varying the types of cations in ionic liquids. The types of cations are noted in the figure and the strain values were measured at a cycle time of 10 s. Figure 3a shows the peak-to-peak displacement ( δ p ) along with the strain ( ε p ) of the actuator comprising P17(75) and [HMIm][PF 6 ], measured with alternating square-wave voltages ranging from ±1 to ±3 V at frequencies of 0.5, 0.05 and 0.025 Hz. As clearly seen from the figure, the degree of electromechanical deformation was roughly proportional to the applied voltage, signalling the absence of faradaic reactions [33] . The actuator also displayed fast restoration motion at a negative potential, suggesting that reversible and fast ion motions resulted from a given stimulus with structural/chemical integrity. The highest generated strain achieved in the present study was ε p =4% (at ±3 V). Most importantly, large δ p -values of 1.4–2.4 mm were attained in the frequency range of 0.025–0.5 Hz at ±1 V, which exceeded the best performance of other ionic polymer actuators reported to date. Figure 3: Factors affecting the actuation performance. ( a ) Displacement (strain)-frequency-voltage dependency of the actuator comprising P17(75) and [HMIm][PF 6 ] measured with alternating square-wave voltages. ( b ) Peak-to-peak strain values of the actuators comprising P17(75) and ionic liquids, compared with those of PVdF-HFP and ionic liquids, by varying the types of cations in ionic liquids. The types of cations are noted in the figure and the strain values were measured at a cycle time of 10 s. Full size image When the type of cations in ionic liquids was varied from [HMIm] to [EMIm] while keeping the same [PF 6 ] anion, based on the anticipation that the cations do have much effect on the charging behaviour, the strain dropped by more than one third for the same ionic liquid loadings (60 wt%). Representative data shown in Fig. 3b were obtained for the actuator comprising P17(75) copolymer, measured at±3 V with a cycle time of 10 s. Such a behaviour was consistently observed for other actuators fabricated with P17(20) and P17(30) copolymers. This should be due, in part, to the relatively small van der Waals volume of the [EMIm] cations. We also observed a 20-fold decrease in conductivity with [EMIm][PF 6 ] compared with [HMIm][PF 6 ] (data are given in Supplementary Fig. S3 ), indicating that much enhanced ion conduction occurred within the [HMIm][PF 6 ]-containing polymer matrix, although the diffusion coefficient of [HMIm] is known to be lower than that of [EMIm] for neat ionic liquids [46] . We can thus infer that the ion transport properties of polymer electrolytes integrated with ionic liquids are not necessarily associated with the intrinsic properties of the ionic liquids but are dominated by the ionic interaction among ionic moieties [47] . The 0-K binding energies of ion pairs are listed in Table 1 (their coupling schemes are given in Supplementary Fig. S4 ). The increase in the length of alkyl substituent in imidazolium was found to cause a small but noticeable reduction in the strength of the ionic interaction between cations and counterions. As the PF 6 − anion was weakly bound to the cations compared with the −SO 3 − anion, the [−SO 3 H] groups that were localized within the ionic PSS phases of the HEX structure would result in effective dissociation of the ionic liquids. To evaluate the performance of our actuators, a conventional poly(vinylidene fluoride- co -hexafluoropropylene) (PVdF-HFP) copolymer (Kynar Flex 2801, random copolymer) was employed as a benchmark material. As shown in Fig. 3b , our actuators showed an eightfold increase in strain when compared with the actuators comprising state-of-the-art PVdF-HFP and the same type and amount of ionic liquids. Although a concrete interpretation of dissimilar bending performance of two different systems may be complicated by multiple factors, the higher conductivity obtained for the P17(75) than PVdF-HFP should be noted (see Supplementary Fig. S3 ). This implies that the creation of well-defined ionic channels within the self-assembled polymer matrix was beneficial for achieving improved bending performance owing to the formation of less tortuous ion pathways facilitating fast and efficient ion transport across the polymer layers [43] , [48] . In particular, the confinement of ions within nanoscale channels leads to the increment of the local concentration of ions, lowering of the activation barrier for ion conduction because of the close proximity of ions [49] . Low-voltage-driven actuators As the focus of the present study is to develop low-voltage-driven actuators, we explored the possible application of our systems to these actuators by monitoring the bending motion below 1 V at frequency range of 0.05–10 Hz. 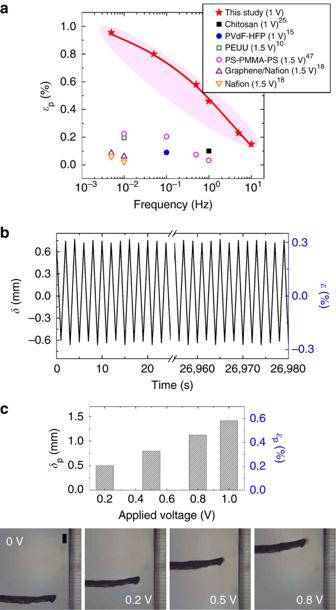Figure 4: Low-voltage-driven actuators. (a) Strain-frequency-voltage dependency of the actuator comprising P17(75) copolymer and [HMIm][PF6], compared with those reported in literatures with a focus on low-voltage operation. (b) Cycle life of the actuator strip (6 mm in length, 1 mm in width, 70 μm in thickness) under continuous operation in air at alternating square-wave voltages of ±1.0 V with a frequency of 0.5 Hz. (c) Actuation performance obtained at sub-1-V conditions and a series of photographs taken at the tip position of the actuator strip every 1 s with step changes in voltage from 0 to 0.2, 0 to 0.5 and 0 to 0.8 V. The line patterns in the photographs were fabricated by microcontact printing with a polydimethylsiloxane (PDMS) stamp; scale bar, 100 μm. Figure 4a shows the strain-frequency dependency of the actuator composed of the P17(75) copolymer and 60 wt% [HMIm][PF 6 ] compared with the values reported in the literatures. The actuation properties distinctly deviated from the trend line, that is, large ε p -values of 0.5–1.0% ( δ p =1.2–2.1 mm) were recorded at ±1 V in the frequency range of 0.05–1 Hz, which marked significant progress from the previously reported results. Upon further increasing the frequency from 1 to 10 Hz, although deterioration in the bending response was observed, the actuation performance was still notable. For example, at 1 V the actuator strip moved 0.3 mm within 0.1 s and then reached to a displacement of 1.2 mm in 1 s, suggesting that the actuator could be successfully operated with a small battery. Supplementary Movie 1 demonstrates the fast motion of our actuators recorded at alternating square-wave voltages of±1 V and a frequency of 1 Hz. Figure 4: Low-voltage-driven actuators. ( a ) Strain-frequency-voltage dependency of the actuator comprising P17(75) copolymer and [HMIm][PF 6 ], compared with those reported in literatures with a focus on low-voltage operation. ( b ) Cycle life of the actuator strip (6 mm in length, 1 mm in width, 70 μm in thickness) under continuous operation in air at alternating square-wave voltages of ±1.0 V with a frequency of 0.5 Hz. ( c ) Actuation performance obtained at sub-1-V conditions and a series of photographs taken at the tip position of the actuator strip every 1 s with step changes in voltage from 0 to 0.2, 0 to 0.5 and 0 to 0.8 V. The line patterns in the photographs were fabricated by microcontact printing with a polydimethylsiloxane (PDMS) stamp; scale bar, 100 μm. Full size image In Supplementary Fig. S5 , we have presented a three-dimensional cube summarizing the strain-frequency voltage dependence of our actuators against other ionic polymer actuators reported in the literatures, which clearly illustrates the impact of our results on the structure of future ionic polymer actuators fabricated with ionic liquids. The sub-1-V actuation performance of ionic polymer metal composites actuators is also plotted in Supplementary Fig. S6 , in comparison with the new actuator developed in this study. The new actuators have long-term durability besides their large strains and fast switching response. Figure 4b shows the cycle life in response to ±1.0 V square wave input signals at a frequency of 0.5 Hz; the actuation was repeated over 13,500 cycles in air with negligible changes in the actuator stroke. The successful operation of our actuators at 1 V has motivated us to explore their performance at sub-1-V conditions geared towards biomimetic technologies for micropower sources. As shown in Fig. 4c , the displacement was again found to be linearly proportional to the applied voltage. Even at an applied voltage of 0.2 V, a δ p of 0.5 mm was seen at a cycle time of 2 s for the actuator consisting of P17(75)/[HMIm][PF 6 ]. To the best of our knowledge, this level of low-voltage-driven actuation performance with rapid response has never been reported in the literature. We further explore the applicability of the new actuators in printing-based miniaturized mechanical devices [50] . We fabricate 50-μm line patterns using microcontact printing with a polydimethylsiloxane stamp, and step changes in voltage from 0 to 0.2, 0 to 0.5 and 0 to 0.8 V were applied to the actuator. A series of photographs are taken at the tip position of the actuator strip every 1 s after changing the voltage. The photographs in Fig. 4c display the fast and controlled movements of the actuators in steps of a few hundred microns, which suggested their possible use in cutting-edge technologies, such as biomedical microdevices and microsensors. The versatile use of the actuators in robotics was also explored by shaping the actuators like artificial fingers; the versatility is validated when the fingers spread over a plastic ball, successfully grasping it ( Supplementary Movie 2 ). To investigate the reason behind the improved electromechanical deformation of the actuator comprising nanostructured PSS-b-PMB copolymers, we conducted in-situ SAXS experiments on the actuators upon applying activation fields. The schematic drawing of the measurement setup is given in Fig. 5a . For accurate analysis, we fabricated relatively thick actuators containing a 180-μm thick polymer layer sandwiched between SWCNTs electrodes. The cross-sectional area of the polymer layer was divided into three regions, marked as I (near cathode), II (centre) and III (near anode), and the X-ray beam was transmitted to each region. This experiment was motivated by the fact that although many publications proposed the actuation mechanism of ionic polymer actuators on the basis of their asymmetric swelling and shrinkage [8] , [9] , there have been no systematic studies identifying the exact nature of polymer layers in response to the actuation field. 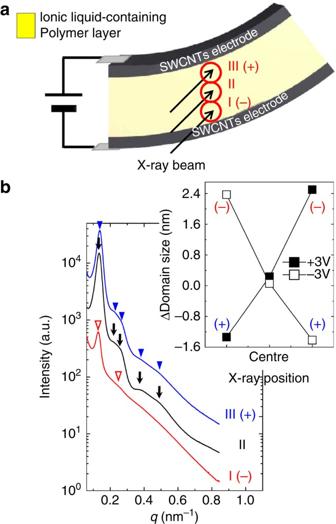Figure 5: Internal structure of the polymer layer during actuation. (a) A schematic drawing of the measurement set-up ofin-situSAXS experiments. (b) Representative SAXS profiles obtained with the actuator comprising P17(75) and [HMIm][PF6], acquired in regions I, II and III under voltages of ±3 V. The change in domain size of the HEX structure in each region upon switching the direction of the applied voltage is plotted in the inset figure. Figure 5: Internal structure of the polymer layer during actuation. ( a ) A schematic drawing of the measurement set-up of in-situ SAXS experiments. ( b ) Representative SAXS profiles obtained with the actuator comprising P17(75) and [HMIm][PF 6 ], acquired in regions I, II and III under voltages of ±3 V. The change in domain size of the HEX structure in each region upon switching the direction of the applied voltage is plotted in the inset figure. Full size image Representative SAXS profiles of the actuator comprising P17(75) and 60 wt% [HMIm][PF 6 ], acquired in each region after 30 min under a voltage of ±3 V, are shown in Fig. 5b . Non-significant changes in the HEX morphology and domain size were observed at the centre of the polymer layer (region II) signalling that the net movement of ions was offset. In contrast, the morphology monitored near the cathode (region I) was significantly disrupted, as shown by the broad Bragg peak and the loss of long-range order. This indicates that the segregation strength between the ionic PSS domains and PMB phases was reduced because of the dominant steric repulsion among excessive [HMIm] cations within the PSS domains. In region III, the HEX morphology was less disturbed, with preserved high-order Bragg reflections. The change in the domain size of the HEX structure in each region is plotted in the inset figure of Fig. 5b . An increase in domain size as large as 2.4 nm was detected near the cathode, contrary to the relatively small decrease of 1.4 nm near the anode. These changes were observed repeatedly upon switching the direction of the applied voltage, as noted in the figure. These dimensional gradients created in the polymer layer should stem from the predominant migration of [HMIm] cations along the well-connected ionic channels. We believe the development of such unique internal structures in the polymer layer stimulated the fast bending response. On the basis of the results obtained so far, the proposed actuation mechanism in the actuators comprising nanostructured block copolymers and ionic liquids is illustrated schematically in Fig. 6 . When a voltage was applied between the two electrodes, the fast electromechanical deformation of the actuator was driven by the rapid creation of dimensional gradients within the polymer layer, which was responsible for their fast sub-1-V switching response. The bending motion of the actuators is continued by the electric charging and discharging at SWCNTs electrodes with non-detectable back relaxation behaviour. Note that the expansion and shrinkage of the electrodes as a result of ion migration are omitted in the drawing for clarity. Intriguingly, the unique internal structure of the polymer layer developed just after applying the voltage is found to be unchanged during the actuation, as monitored by in-situ SAXS. This is quite surprising, as the formation of electric double layer at the interface of the electrode and the polymer layer would result in the removal of electric potential gradient in the polymer layer. We infer that relatively high glass transition temperature ( T g ) of the PSS-b-PMB block copolymers containing ionic liquids, ca. 60 °C, slows down the self-relaxation of ions in the absence of external stimuli. The observed actuation performance may be further tuned by varying the type of ionic liquids and by employing a range of PSS-b-PMB copolymers with different molecular weights and compositions. Experiments on whether the morphology effects are present in the actuators will be a subject of our future studies. Further improvement of actuation performance by optimizing the types of electrode is currently underway. 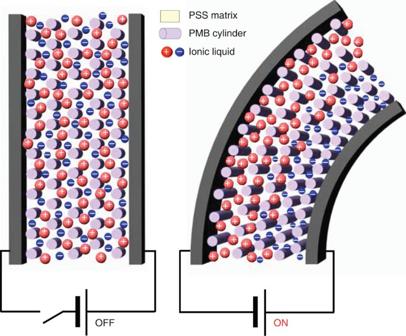Figure 6: Actuation mechanism in our actuator. Schematic illustration of the internal structure of the actuator as a result of actuation. The creation of dimensional gradients within the polymer layer was responsible for the fast and efficient electromechanical deformation of the actuator. Figure 6: Actuation mechanism in our actuator. Schematic illustration of the internal structure of the actuator as a result of actuation. The creation of dimensional gradients within the polymer layer was responsible for the fast and efficient electromechanical deformation of the actuator. Full size image We conclude this paper by commenting on the impact of our work on the structure of widely studied ionic polymer actuators. The use of nanostructured sulphonated block copolymers integrated with ionic liquids in actuators enables us to achieve largely improved actuation performance without any signs of back relaxation by offering fast and efficient ion transport across the polymer layers. By comparing the strain-frequency voltage dependence of our actuators against other ionic polymer actuators reported to date, it became further evident that the actuation properties of our actuators exceeded the best reported performance of the other actuators. The new actuators also demonstrate outstanding functionality at high frequency and sub-1-V conditions, with negligible changes in the actuator stroke over 13,500 cycles in air. The organized ion migration along well-connected ionic channels is confirmed by observations of the internal structure of polymer layers during actuation, which enables the rapid actuation response of our actuators. Our results confirm that the nanostructured block copolymer electrolytes with tailored ionic interactions allow the successful actuator operation with a small battery, which paves the way for more advanced biomimetic technologies in the future. Synthesis of ionic block copolymers A poly(styrene-b-methylbutylene) (PS-b-PMB, 16.8–18.7 kg mol −1 ) copolymer was synthesized by sequential anionic polymerization of styrene and isoprene monomers followed by selective hydrogenation of isoprene units [51] . The molecular weight and molecular weight distribution of the PS-b-PMB copolymer were characterized by combining 1 H-NMR (Bruker AVB-300) spectroscopy and gel permeation chromatography (Waters Breeze 2 HPLC). The polydispersity index of the PS-b-PMB copolymer was 1.03, measured on gel permeation chromatography with polystyrene standards in tetrahydrofuran (THF) for calibration. The styrene chains of PS-b-PMB copolymer were then partially sulphonated using procedures described in ref. 51 , which were referred to as PSS-b-PMB block copolymers. Samples with different SL were prepared by controlling reaction time; SL=20 mol% with 0.3 h reaction, SL=30 mol% with 0.5 h reaction and SL=75 mol% with 30 h reaction. Characterization of PSS-b-PMB block copolymers PSS-b-PMB films were cryomicrotomed at −120 °C to obtain thin sections with thicknesses in the 80–120 nm range using an RMC Boeckeler PT XL Ultramicrotome. The electron contrast in the samples was enhanced by exposure to ruthenium tetroxide (RuO 4 ) vapour for 50 min. Transmission electron micrographs on stained samples were obtained with a Hitach H-800 microscope operating at 100 kV. The Young’s moduli of the PSS-PMB films were measured from load-displacement curves using depth-sensing nano-indentation (Nano indenter XP II, MTS Corp.). For accurate measurements of soft polymer films, a dynamic contact module with improved resolution in displacement and load was used. Ionic liquids [EMIm][BF 4 ], ≥98% HPLC grade, [EMIm][PF 6 ],≥97% HPLC grade and [HMIm][PF 6 ], ≥97% HPLC grade were purchased from Sigma-Aldrich and used as received. Preparation of actuators SWCNTs produced by a CoMoCAT catalytic CVD process were purchased from Sigma-Aldrich and used without further purification. To prepare SWCNTs electrodes, 82 mg of [EMIm][BF 4 ], 50 mg of PVdF-HFP (Kynar Flex 2801, Arkema Chemical Inc.) and 33 mg of SWCNTs were dissolved in 6 ml of N , N -dimethylacetamide (≥99.9% HPLC grade, Sigma-Aldrich). The mixture was stirred at room temperature for 24 h and placed in an ultrasonic bath for 6 h. The electrode layer was fabricated by casting the mixture onto a Teflon plate (2 cm × 2 cm) at room temperature, followed by vacuum drying at 80 °C. The thickness of the obtained electrode film was 20–30 μm. Note that [PF 6 ]-containing ionic liquids were not used for the fabrication of SWCNT electrodes because of the poor interfacial properties between the electrode and the polymer layer, which appeared to cause a significant deterioration in the actuator properties, that is, decreased displacements and slow response times. For the preparation of polymer layers, inhibitor-free anhydrous THF (≥99.9%) and degassed methanol were used. THF is a neutral good solvent for both PSS and PMB chains, whereas MeOH is a PSS-selective one. Predetermined quantities of PSS-b-PMB copolymers and ionic liquids were weighed into vials and ~5 wt% solutions were prepared using 80/20 vol% THF and methanol mixtures, which appeared to be an ideal composition to obtain highly ordered nanostructures where the use of MeOH allows the selective incorporation of ionic liquids within PSS phases. One-hundred-micrometre-thick membranes were prepared by solvent casting onto an aluminum mold (an area of 1 cm × 1.5 cm) at room temperature under an argon atmosphere for 2 days followed by vacuum drying at 70 °C for 7 days. The dried polymer membrane was subjected to a normal stress of about 200 kgf cm −2 in a hydraulic Carver press at 25 °C for 12 h to yield dominant parallel orientation of hexagonal cylinder microdomains [51] , [52] . The polymer membranes were then sandwiched between two SWCNTs electrodes via hot pressing, which yields a monolithic trilaminar structure. Rectangular pieces (8 mm × 1 mm) were cut from the membrane and the final structure of the actuator was examined by SEM (a Helios Nanolab 600) with a 5-keV accelerating voltage. Representative cross-sectional SEM image is given in Supplementary Fig. S1 . Actuator performance tests The 8 mm × 1 mm-sized actuator strips were clipped by two Pt disk electrodes yielding 6-mm free length from Pt contacts. Actuator performance were tested by applying square wave voltages to the actuator strips using a function generator (FG-1880B, ED Corp.) and an oscilloscope (DSP3202A, Aglient Technologies Inc.). The time-dependent bending motion of the actuators under given applied voltages was recorded using a Zeiss microscope (AxioVision) equipped with a charge-coupled device camera. The displacement ( δ ) of the actuator was measured using image-processing software, which was transformed into the strain ( ε ) using the following equation [14] : where L is the free length from Pt contacts and d is the thickness of actuator. All measurements were carried out under ambient lab atmosphere, where the average relative humidity (RH) is recorded as RH=20±5%. Conductivity measurements The conductivity of PSS-b-PMB copolymers integrated with ionic liquids was measured by combining a potentiostat (PARSTAT 2273) and an AC impedance spectroscopy (Solartron 1260). The conductivity was measured using a home-built two-electrode cell with 1.25 cm × 1.25 cm stainless steel blocking electrodes and 1 cm × 1 cm Pt working/counter electrodes. Data were collected over a frequency range of 1–100,000 Hz. In-situ synchrotron SAXS In-situ SAXS measurements on the actuators were performed using the PLS-II 9A U-SAXS beam-line at the Pohang Accelerator Laboratory equipped with the function generator and the oscilloscope. The X-ray beam size at the sample position was as small as 60 μm and the sample was mounted on the motorized seven-axis sample stage for the fine alignment in ±1.0 μm step. This is to examine different sample areas beneath the cathode during actuation. The wavelength ( λ ) of the incident X-ray beam was 0.1115, nm (Δ λ / λ =2 × 10 −4 ) and sample-to-detector distance of 4.5 m was used yielding scattering wave vector q ( q =4 π sin( θ /2)/ λ , where θ is the scattering angle) in the range 0.04–1.03 nm −1 . The resulting scattering data were collected using 2D CCD detector (Rayonix SX165, USA) and averaged azimuthally to obtain scattering intensity versus q . How to cite this article: Kim, O. et al. Fast low-voltage electroactive actuators using nanostructured polymer electrolytes. Nat. Commun. 4:2208 doi: 10.1038/ncomms3208 (2013).